Understanding complete oxidation of methane on spinel oxides at a molecular level It is crucial to develop a catalyst made of earth-abundant elements highly active for a complete oxidation of methane at a relatively low temperature. NiCo 2 O 4 consisting of earth-abundant elements which can completely oxidize methane in the temperature range of 350–550 °C. Being a cost-effective catalyst, NiCo 2 O 4 exhibits activity higher than precious-metal-based catalysts. Here we report that the higher catalytic activity at the relatively low temperature results from the integration of nickel cations, cobalt cations and surface lattice oxygen atoms/oxygen vacancies at the atomic scale. In situ studies of complete oxidation of methane on NiCo 2 O 4 and theoretical simulations show that methane dissociates to methyl on nickel cations and then couple with surface lattice oxygen atoms to form –CH 3 O with a following dehydrogenation to −CH 2 O; a following oxidative dehydrogenation forms CHO; CHO is transformed to product molecules through two different sub-pathways including dehydrogenation of OCHO and CO oxidation. A complete oxidation of hydrocarbons has been a significant topic in the field of heterogeneous catalysis for decades since unburned hydrocarbons must be transformed in power plants or before release of gas exhaust from various engines of vehicles using gasoline, diesel, natural gas or liquid petroleum gas (a mixture of propane, isobutene, n -butane and ethane). Thermal stability of a catalyst (for removal of CH 4 or other hydrocarbons) at a temperature of 1,300 °C for applications to power plants or at least 800 °C for engines using gasoline or diesel is requested. Ying et al . reported that CeO 2 nanoparticles supported on barium hexaaluminate exhibits high activity at a quite high temperature and remains its structure up to 1,300 °C (ref. 1 ). Recently, Gorte, Fornasiero, and Farrauto and their coworkers reported that a catalyst of Pd nanoparticles caged in a porous CeO 2 shell supported on Al 2 O 3 exhibits exceptionally high activity for a complete oxidation of methane with a high thermal stability up to 850 °C (refs 2 , 3 ). The activity of Co 3− x Cu x O 4 , Co 3− x Zn x O 4 , and Co 3− x Ni x O 4 for oxidation of hydrocarbons was reported in 1968 and the following studies [4] , [5] , [6] , [7] . A very recent study showed the high activity of these oxides in oxidation of (a) a mixture of liquefied petroleum gas and CO or (b) a liquefied petroleum gas without CO [8] . Use of natural gas vehicles is a programme launched in Europe and other countries towards diversity of energy sources and utilization of methane, the inexpensive, earth-abundant energy sources [9] , [10] , [11] , [12] . The exhaust of natural gas engines has the following features [9] : low temperature (<500–550 °C), low CH 4 concentration (about 1,000 p.p.m. ), large amount of water vapour (10%), high O 2 :CH 4 ratio, and presence of NO x or SO x (refs 9 , 12 ). A complete oxidation of methane at a relatively low temperature (<500–550 °C) is critical for abating unburned methane of the exhaust of engines of natural gas vehicles [9] , [11] , [12] , [13] . Pt and Pd supported on Al 2 O 3 are the well-studied catalysts [9] . Significant efforts have been made in fundamental understanding of mechanism of the complete oxidation of methane [14] and optimization of catalytic performances of these Pt- or Pd-based catalysts [9] . From reaction mechanism point of view, Neurock and Iglesia et al . first elucidated the reaction mechanism on Pd-based catalysts at a molecular level [14] ; these Pd-based catalysts exhibit different mechanisms of activation of C–H along increase of chemical potential of oxygen. The high cost of precious metals has driven the search of catalysts made of earth-abundant elements. Spinel oxide, a type of reducible early transition metal oxides, consists of M 2+ and M 3+ in its lattice. Co 3 O 4 is one of the spinel oxides. It has almost weakest M–O bonds among all transition metal oxides [15] , [16] . Oxygen vacancies can be readily generated even at a temperature below 25 °C (refs 17 , 18 ). In addition, the barrier for hopping oxygen vacancies on the surface of Co 3 O 4 is only 0.23 eV (ref. 17 ). Due to the high density of oxygen vacancies of surface of Co 3 O 4 (refs 15 , 19 ), Ni cations and oxygen vacancies are mixed at atomic scale, while Ni cations are integrated to the lattice of Co 3 O 4 through formation of a doped spinel oxide Ni x Co 3− x O 4 . 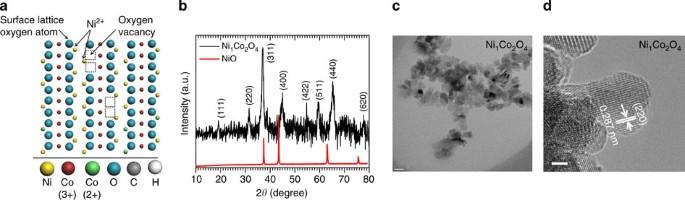Figure 1: NiCo2O4catalyst for a complete oxidation of methane. (a) Schematic showing a surface of NiCo2O4catalyst. (b) XRD pattern of NiCo2O4catalyst. (c) Large-scale TEM image; scale bar, 10 nm. (d) High-resolution TEM image; scale bar, 2 nm. Figure 1a schematically shows the integration of Ni cations, Co cations and surface lattice oxygen atoms and vacancies at atomic scale. Although catalytic activity of a complete oxidation of hydrocarbons on doped cobalt oxides was reported as early as 1968 (refs 4 , 5 , 6 , 7 , 8 ), there is lack of mechanistic understanding of the complete oxidation of hydrocarbons at a molecular level. Compared with the well-studied complete oxidation of CH 4 on Pt or Pd-based catalysts [9] , the complete oxidation on NiCo 2 O 4 could fellow a different mechanism. Figure 1: NiCo 2 O 4 catalyst for a complete oxidation of methane. ( a ) Schematic showing a surface of NiCo 2 O 4 catalyst. ( b ) XRD pattern of NiCo 2 O 4 catalyst. ( c ) Large-scale TEM image; scale bar, 10 nm. ( d ) High-resolution TEM image; scale bar, 2 nm. Full size image Here we focus on mechanistic exploration of a complete oxidation of methane on NiCo 2 O 4 at a molecular level. Multiple in situ techniques are used in experimental exploration of the catalytic mechanism. Surface chemistry of this mixed oxide during catalysis is tracked with ambient pressure X-ray photoelectron spectroscopy (AP-XPS) [20] . Vibrational signature of surface adsorbates is identified with in situ infrared spectroscopy. In addition, computational studies for understanding of the mechanism of the complete oxidation of methane on NiCo 2 O 4 at a molecular scale are performed. Catalytic performance for complete oxidation of CH 4 Catalyst NiCo 2 O 4 was synthesized with a coprecipitation method described in the section of Methods. X-ray diffraction ( Fig. 1b ) showed that NiCo 2 O 4 nanoparticles have the same spinel structure as Co 3 O 4 . NiCo 2 O 4 catalyst consists of nanoparticles with a size of 3–6 nm (transmission electron microscopic (TEM) images; Fig. 1c,d ). With the same method, Ni 0.75 Co 2.25 O 4 and Ni 1.25 Co 1.75 O 4 were prepared. X-ray diffraction and TEM studies confirmed the formation of lattice of spinel oxide ( Supplementary Figures 1 and 2 , and Supplementary Methods ). Catalytic performances of a complete oxidation of CH 4 on these catalysts were measured in a fixed-bed flow reactor. Certain amount of a catalyst given in figure captions was used in different experiments. 10% CH 4 balanced with Ar, and 99.99% O 2 , and 99.99% Ar with certain flow rates were mixed and then flowed through a catalyst bed. The molar ratio of the introduced CH 4 and O 2 is 1:5 for all experiments in Fig. 2 . NiCo 2 O 4 is extraordinarily active in combustion of CH 4 to CO 2 and H 2 O. CH 4 is completely combusted at 350 °C, while gas hourly space velocity (GHSV) of methane is 24,000 ml 5% CH 4 g −1 h −1 ( Fig. 2 ). At the same GHSV, pure Co 3 O 4 and pure commercial NiO with surface areas similar to NiCo 2 O 4 exhibit a conversion of only 8% and 0% at 350 °C, respectively ( Fig. 2 ). The pure Co 3 O 4 without any Ni cations exhibits a much lower conversion than NiCo 2 O 4 though it has the same lattice of a spinel structure. This distinct difference in catalytic performance between NiCo 2 O 4 and pure Co 3 O 4 in the temperature range of 200–425 °C shows that Ni cations are crucial sites for dissociation of CH 4 , which was supported by experimental studies and theoretical findings in the following sections. The catalytic performance of complete combustion at 350 °C is remained even after heating to 550 °C and then cooling to 200 °C ( Fig. 3a ). Kinetic studies were performed in the temperature range of 270–330 °C, while catalysis was in a kinetics control regime by controlling conversions <10%. The measured activation barrier is about 108 kJ mol −1 ( Supplementary Fig. 3 ). In addition, NiCo 2 O 4 exhibits durability in complete oxidation of methane at 350 °C and 550 °C for over 48 h ( Fig. 3b,c ). The thermal stability of catalyst structure was confirmed by the preservation of X-ray diffraction pattern of NiCo 2 O 4 after a complete oxidation at 550 °C ( Supplementary Fig. 4 ). In addition, NiCo 2 O 4 remains the original particle size after a complete oxidation at 550 °C as shown in Supplementary Fig. 5 . This is consistent with the thermal stability of NiCo 2 O 4 suggested by the thermal analysis of coprecipitated products and NiCo 2 O 4 (ref. 21 ). 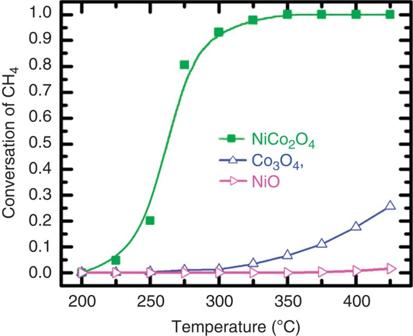Figure 2: Conversion of CH4. Conversion of CH4in a complete oxidation of CH4on NiCo2O4in the temperature range of 200–425 °C . The gas composition of the feed gas is 5% CH4, 25% O2and 70% Ar. Molar ratio of CH4to O2in the gas mixture is always 1:5. As 500 mg NiCo2O4catalyst was used, the GHSV of CH4is 24,000 ml 5% CH4g−1h−1; at this GHSV the conversion of CH4on NiCo2O4at 350 °C is 100%. Figure 2: Conversion of CH 4 . Conversion of CH 4 in a complete oxidation of CH 4 on NiCo 2 O 4 in the temperature range of 200–425 °C . The gas composition of the feed gas is 5% CH 4 , 25% O 2 and 70% Ar. Molar ratio of CH 4 to O 2 in the gas mixture is always 1:5. As 500 mg NiCo 2 O 4 catalyst was used, the GHSV of CH 4 is 24,000 ml 5% CH 4 g −1 h −1 ; at this GHSV the conversion of CH 4 on NiCo 2 O 4 at 350 °C is 100%. 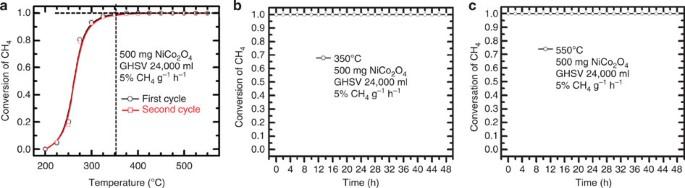Figure 3: Catalytic performances of NiCo2O4in the temperature range of 200–550 °C. (a) CH4can be completely oxidized at a temperature up to 550 °C (black line), and the catalytic performance remains the same after heating to 550 °C and then cooling to 200 °C (red line). (b) Conversion of a complete oxidation of CH4on NiCo2O4at 350 °C for 48 h. (c) Conversion of a complete oxidation of CH4on NiCo2O4at 550 °C for 48 h. Full size image Figure 3: Catalytic performances of NiCo 2 O 4 in the temperature range of 200–550 °C. ( a ) CH 4 can be completely oxidized at a temperature up to 550 °C (black line), and the catalytic performance remains the same after heating to 550 °C and then cooling to 200 °C (red line). ( b ) Conversion of a complete oxidation of CH 4 on NiCo 2 O 4 at 350 °C for 48 h. ( c ) Conversion of a complete oxidation of CH 4 on NiCo 2 O 4 at 550 °C for 48 h. Full size image Surface chemistry of NiCo 2 O 4 during catalysis Measurements of bulk composition of NiCo 2 O 4 catalyst using inductively coupled plasma Auger electron spectroscopy show that atomic ratio of Ni and Co in bulk of the NiCo 2 O 4 nanoparticles is 1:2. Similar to the obvious difference in composition of bimetallic nanoparticle between surface and bulk [22] , the difference in atomic ratio of Ni/Co of NiCo 2 O 4 catalyst between surface and bulk was uncovered here as well. To achieve a deep understanding of the complete oxidation of methane on NiCo 2 O 4 , we performed in situ studies using AP-XPS [15] , [20] , [23] , [24] in the temperature range of 60–400 °C by following the reaction conditions used for measurements of catalytic performances in a fixed-bed flow reactor. Surface chemistry of NiCo 2 O 4 (a) in UHV, (b) in a reactant gas (CH 4 or O 2 ) at room temperature, (c) in a mixture of reactant gases (CH 4 +O 2 ) at room temperature and (d) in a mixture of reactant gases (CH 4 +O 2 ) in the temperature range of 25–400 °C were studied. Photoemission features of Co 2 p , Ni 2 p , and O 1 s of NiCo 2 O 4 collected under conditions (a), (b) and (c) are quite similar; in addition, the atomic ratios of O/(Ni+Co) of the catalyst surface under the three conditions are the same. However, the atomic ratio O/(Ni+Co) in the gaseous environment of CH 4 and O 2 exhibits a temperature-dependent evolution which will be discussed in the following paragraphs. During the data acquisition of in situ studies, NiCo 2 O 4 catalyst was remained in a mixture of CH 4 and O 2 (molar ratio 1:5) in Torr pressure range. 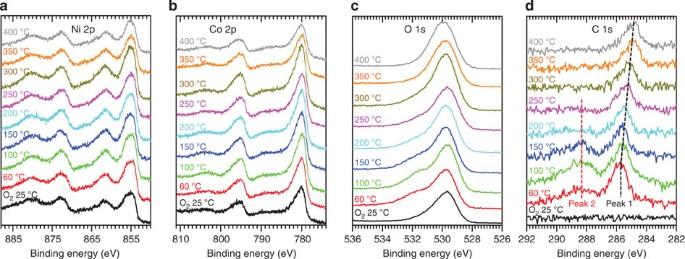Figure 4: Photoemission features. Photoemission features of NiCo2O4at different temperatures during catalysis on NiCo2O4in CH4and O2with a molar ratio of 1:5 at Torr pressure range. (a) Ni 2p, (b) Co 2p, (c) O 1s, and (d) C 1s. Figure 4 , Supplementary Fig. 6 and Supplementary Fig. 7 present photoemission features of NiCo 2 O 4 , Ni 0.75 Co 2.25 O 4 and Ni 1.25 Co 1.75 O 4 during catalysis, respectively. As shown in Fig. 4a,b , the photoemission features of Ni 2 p and Co 2 p remain constant in the temperature ranges of 60–400 °C. Surprisingly, two C 1 s peaks at 285.6 eV (peak 1) and 288.3 (peak 2) were clearly observed even at 60 °C ( Fig. 4d ). 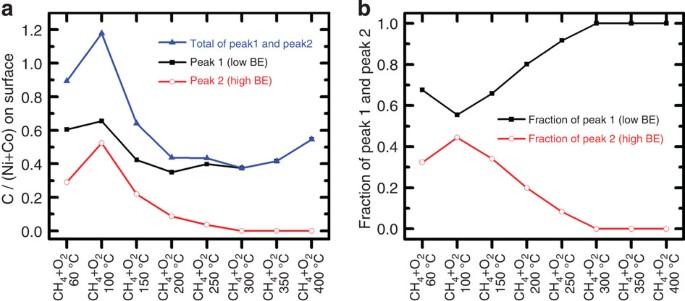Figure 5: Evolution of surface concentration of carbon-containing species. Evolution of surface concentration of carbon-containing species during catalysis at different temperature based onin situstudies of NiCo2O4surface by AP-XPS. (a) Atomic ratio of,, andand (b) atomic fraction of carbon species 1 (peak 1),and carbon species 2 (peak 2),at different temperatures. The error of measurement of peak area is ±5% of the corresponding peak area. Figure 5a shows the evolution of the surface atomic ratio, of the two C 1 s peaks of Fig. 4d along the increase of catalysis temperature. One interesting evolution is a quick increase of species 2 (peak 2 in Fig. 4d ), a following decrease, and then a nearly complete disappearance of this species at about 250 °C (red lines in Fig. 5a,b ) where the conversion of CH 4 starts to increase largely ( Fig. 2 ). The sharp decrease of on NiCo 2 O 4 (red line in Fig. 5a ) and a following decrease and then disappearance at 250–300 °C along the rapid increase of catalytic conversion at 250–300 °C (green line in Fig. 2 ) suggests species 2 (peak 2 in Fig. 4d ) is an intermediate in the formation of CO 2 molecules. Figure 4: Photoemission features. Photoemission features of NiCo 2 O 4 at different temperatures during catalysis on NiCo 2 O 4 in CH 4 and O 2 with a molar ratio of 1:5 at Torr pressure range. ( a ) Ni 2 p , ( b ) Co 2 p , ( c ) O 1 s , and ( d ) C 1 s . Full size image Figure 5: Evolution of surface concentration of carbon-containing species. Evolution of surface concentration of carbon-containing species during catalysis at different temperature based on in situ studies of NiCo 2 O 4 surface by AP-XPS. ( a ) Atomic ratio of , , and and ( b ) atomic fraction of carbon species 1 (peak 1), and carbon species 2 (peak 2), at different temperatures. The error of measurement of peak area is ±5% of the corresponding peak area. Full size image In situ infrared studies of catalysts helped assign the two species corresponding to peaks 1 and 2 in Fig. 4d . As shown in Fig. 6 , vibrational peaks at 1,280 1,430 and 1,561 cm −1 were observed in the temperature range of 50–160 °C. Referred to the literature [25] , these vibrational signatures are contributed from formate species (OCHO). The assignment of these vibrational peaks to a formate species is supported by the agreement between C 1 s photoemission peak at 288.3 eV (peak 2 in Fig. 4d ) and 288.5 eV of the reported formate species [25] . Thus, both in situ photoemission feature of C 1 s and in situ vibrational signature of surface species suggest the formation of OCHO species on the surface at a relatively low temperature. C–H vibrational peaks at 2,900–3,000 cm −1 were identified during in situ studies of CH 4 combustion on NiCo 2 O 4 . They are contributed from C–H stretching of the spectator CH n species formed from dissociative adsorption of CH 4 , supported by the low C 1 s binding energy of CH n (peak 1) at 285.9–284.8 eV (refs 25 , 26 , 27 ), and C–H stretching of the intermediate OCHO. 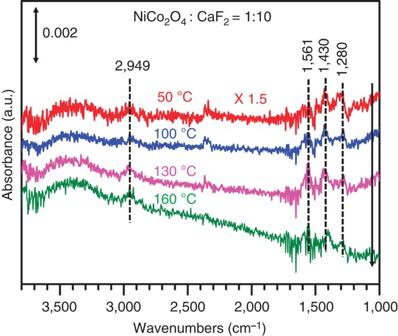Figure 6:In situinfrared studies. In situinfrared studies of the surface species on NiCo2O4catalyst in the mixture with CaF2under the same catalytic condition as the measurement of catalytic performance in a fixed-bed flow reactor. Figure 6: In situ infrared studies. In situ infrared studies of the surface species on NiCo 2 O 4 catalyst in the mixture with CaF 2 under the same catalytic condition as the measurement of catalytic performance in a fixed-bed flow reactor. Full size image To investigate whether that the C 1 s photoemission feature at 284.9–285.8 eV (peak 1 in Fig. 4d ) is assigned to adsorbed CH n species or accumulated atomic carbon of coke, surface of the active catalyst at 400 °C or 140–200 °C in the mixture of CH 4 and O 2 (1:5) was tracked on CH 4 was purged but O 2 kept. The in situ AP-XPS ( Supplementary Fig. 8 ) suggests that the left CH n species on surface at 400 °C reacted with oxygen upon CH 4 was purged and but O 2 remained. As shown in Supplementary Fig. 8 , C 1 s photoemission feature of the left CH n species disappeared within a few minutes due to a quick oxidation by O 2 to form CO 2 . A similar study was designed to test whether the peak 1 of C 1 s spectrum observed at 150 °C in the mixture of CH 4 and O 2 (1:5) ( Fig. 4d ) is coke-like carbon or chemisorbed CH n species. As shown in Supplementary Fig. 9 , these carbon-containing species formed at 140 °C reacted with O 2 to form CO 2 and disappeared at 200 °C in O 2 . Therefore, these designed experiments ( Supplementary Figs 8 and 9 ) suggest that the C1 s at 284.9–285.8 eV (peak 1) is not contributed from accumulated coke-like carbon since a coke-like carbon is not readily oxidized to CO 2 at 400 °C or 140–200 °C (ref. 28 ). Therefore, both C 1 s photoemission feature and C–H vibrational signatures allow us for assigning the carbon-containing species of peak 1 in Fig. 4d to CH n species. It is noted that the coke-like carbon does form by dissociation of CH 4 when NiCo 2 O 4 catalyst is kept in pure CH 4 ( Supplementary Fig. 10d ); in addition, without O 2 , nickel cations of NiCo 2 O 4 are reduced to metallic state at 400 °C ( Supplementary Fig. 10a ); along this reduction, coke-like carbon are formed at 400 °C ( Supplementary Fig. 10d ). It suggests a strong binding of coke-like carbon on metallic Ni atoms [28] . By introducing O 2 to the surface of carbon layers at 400 °C, the C 1 s photoemission feature of coke-like carbon still remains. It further suggests the nature of coke-like carbon formed on NiCo 2 O 4 in the lack of molecular O 2 . By introducing the mixture of CH 4 and O 2 (1:5) to this surface covered with a layer of coke, there is no conversion of CH 4 anymore on it since the catalyst surface has been coved with coke-like carbon. 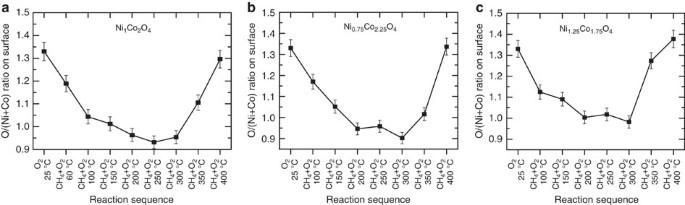Figure 7: Evolution of atomic ratio of oxygen atoms. Evolution of atomic ratio of oxygen atoms to the total of Ni and Co in surface region of three catalysts NiCo2O4(a), Ni0.75Co2.25O4(b) and Ni1.25Co1.75O4(c) along the increase of catalytic temperature during catalysis. The error of measurement of peak area is ±5% of the corresponding peak area. Figure 7a presents the evolution of the surface atomic ratio, along the increase of catalysis temperature of NiCo 2 O 4 . There are two processes involved in the evolution of atom ratio. The formation of OCHO species with a following desorption of CO 2 generates surface oxygen vacancies; an opposite process is the filling of oxygen vacancies with oxygen atoms through dissociation of molecular O 2 . The ‘U’ shape evolution of atomic ratio shows that more oxygen vacancies are created at a medium temperature (150–250 °C). The decrease of the ratio, (namely, the increase of density of oxygen vacancies) at ≤250 °C likely suggests that the formation of oxygen vacancies through desorption of product molecules is relatively faster than filling oxygen vacancies through dissociation of O 2 in this temperature range. At a relatively high temperature such as 300 °C, the atomic ratio starts to increase. It probably results from the accelerated dissociation of O 2 and thus a faster refilling of surface oxygen vacancies (at a higher temperature) than consumption of oxygen atoms through transforming the OCHO intermediate to product molecules CO 2 . The turning point of ratio (about 250 °C) suggests that there is a barrier for O 2 dissociation. For a temperature ≤250 °C, the filling of oxygen vacancies through dissociation of molecular O 2 on oxygen vacancies is kinetically slower than the creation of oxygen vacancies through desorption of intermediate or product molecules; thus, the net outcome is the decrease of ratio at a relatively low temperature. At a relatively high temperature (≥250 °C), however, dissociation of O 2 is accelerated and thus oxygen vacancies are filled rapidly; therefore, the overall consequence is the increase of surface lattice oxygen at a temperature ≥250 °C. Alternatively, a potential oxygen-containing spectator could possibly be formed. It may contribute to the increase of O/(Ni+Co) ratio. Very similar ‘U-shape’ evolution of atomic ratio was observed on Ni 0.75 Co 2.25 O 4 and Ni 1.25 Co 1.75 O 4 ( Fig. 7b,c ) along the increase of the catalysis temperature of complete oxidation of methane. Figure 7: Evolution of atomic ratio of oxygen atoms. Evolution of atomic ratio of oxygen atoms to the total of Ni and Co in surface region of three catalysts NiCo 2 O 4 ( a ), Ni 0.75 Co 2.25 O 4 ( b ) and Ni 1.25 Co 1.75 O 4 ( c ) along the increase of catalytic temperature during catalysis. The error of measurement of peak area is ±5% of the corresponding peak area. Full size image In situ studies using isotope-labelled reactant and catalyst Both in situ AP-XPS and infrared studies have shown the formation of the two species on NiCo 2 O 4 surface in the mixture of CH 4 and O 2 , formate (species 2) and CH n ( n =0–3; species 1). To elucidate the source of oxygen atoms of the intermediate of OCHO species, we performed two temperature programmed reactions using isotope-labelled reactant and isotope-labeled catalyst: (1) CH 4 and on ( Fig. 8a ) and (2) CH 4 and on an isotope-labeled catalyst ( ) ( Fig. 8b ). 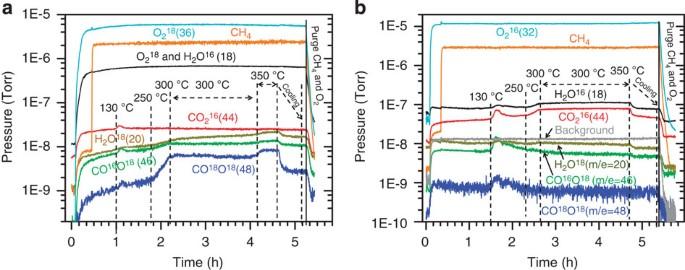Figure 8: Evolution of products. Evolution of products during (a) CH4complete oxidation inon, and (b) CH4complete oxidation inon isotope-labelled catalystalong the increase of catalysis temperature. Figure 8: Evolution of products. Evolution of products during ( a ) CH 4 complete oxidation in on , and ( b ) CH 4 complete oxidation in on isotope-labelled catalyst along the increase of catalysis temperature. Full size image In the complete oxidation of CH 4 in on ( Fig. 8a ), products formed in the reaction cell of the AP-XPS were measured with an on-line mass spectrometer. One of the products, CO 16 O 18 (M/z=46; green line in Fig. 8a ) was clearly observed. The formation of CO 16 O 18 suggests that surface lattice oxygen atoms O 16 of participated into the formation of CO 2 since the reactant gas does not have O 16 atoms. The co-existence of O 16 and O 18 in CO 16 O 18 product suggests that molecular O 2 dissociates on surface during complete oxidation of CH 4 . Another experiment is the CH 4 combustion in on an isotope-labeled catalyst ( Fig. 8b ). The isotope-labeled catalyst was prepared by annealing the catalyst to 350 °C in a flowing . The preparation of was done in an attached high-pressure reactor of AP-XPS system which is different from the reaction cell of AP-XPS since our AP-XPS system has both reaction cell for AP-XPS studies and high-pressure reactor for pretreatment. Upon the preparation, was purged and a UHV environment (3 × 10 −9 torr) was achieved before was transformed to the reaction cell of AP-XPS. Then, combustion of CH 4 was performed on this isotope-labeled catalyst in pure in the reaction cell of AP-XPS. The evolution of partial pressure of the three potential products CO 16 O 16 (M/z=44), CO 16 O 18 (M/z=46), and CO 18 O 18 (M/z=48) were recorded with the mass spectrometer ( Fig. 8b ). It is noted that CO 16 O 18 (M/z=46) was produced even at a relatively low temperature 130–150 °C; However, the partial pressure of CO 16 O 18 (M/z=46) decreased to its base line at a temperature higher than 150 °C. The decrease of CO 16 O 18 partial pressure results from that fact that the source of O 18 atoms in the isotope-labelled catalyst is limited. The observation of CO 16 O 18 shows that the surface lattice oxygen atoms directly participate into the formation of intermediate towards formation of product molecules. Catalytic performance for removal of CH 4 in gas exhaust To examine the catalytic performance of NiCo 2 O 4 in a complete oxidation of CH 4 of gas exhaust of an engine of natural gas, we measured catalytic performance of a complete oxidation of CH 4 on NiCo 2 O 4 in two different mixtures with gas compositions ( Fig. 9 ) similar to the exhaust of lean-burn natural gas engine: (1) CH 4 0.2%, O 2 5%, CO 2 15%, H 2 O 10% balanced with Ar with a flow rate of 200 ml min −1 ( Figs 9a ), and (2) CH 4 0.2%, O 2 5%, NO 0.15%, H 2 O 10% balanced with Ar ( Fig. 9b ). These gas compositions are typically used in the evaluation of catalytic performance of Pd- and Pt-based catalysts for a complete oxidation of CH 4 in the exhaust of engines of natural gas [11] , [12] , [13] . In the mixture of CH 4 0.2%, O 2 5%, CO 2 15% and H 2 O 10%, balanced with Ar, CH 4 can be completely oxidized to CO 2 and H 2 O on 200 mg NiCo 2 O 4 at 425 °C ( Fig. 9a ). Compared with 200 mg of NiCo 2 O 4 , 200 mg of 2.2wt%Pd/Al 2 O 3 can completely oxidize the mixture of 0.2% CH 4 , O 2 5%, CO 2 15% and H 2 O 10% at 500 °C or higher [11] . Thus, NiCo 2 O 4 exhibits higher activity than Pd/Al 2 O 3 in the complete oxidation of CH 4 of exhaust gas in the temperature range of 400–500 °C. In the case of CH 4 0.2%, O 2 5%, NO 0.15% and H 2 O 10% balanced with Ar, CH 4 can be oxidized completely to CO 2 and H 2 O at 475 °C, while 200 mg NiCo 2 O 4 is used ( Fig. 9b ). As the cost of Pd per kg is largely higher than nickel oxide and cobalt oxide by >3,000 times, the cost of raw materials of NiCo 2 O 4 is <1% of the catalyst 2.2wt%Pd/Al 2 O 3 . Thus, NiCo 2 O 4 is more active and certainly cost-effective compared with Pd/Al 2 O 3 or Pt/Al 2 O 3 . 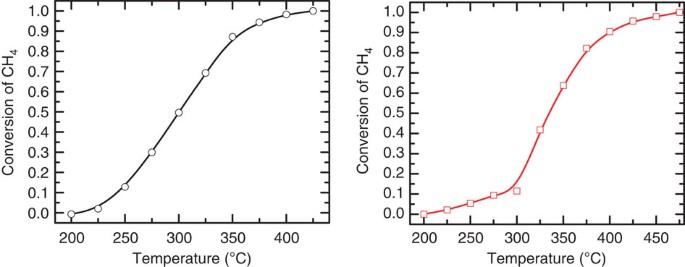Figure 9: Catalytic performance of NiCo2O4in mixture of gases of exhaust of engines of natural gas vehicles. (a) Gas composition, CH4: 0.2%, O2: 5%, CO2: 15%, H2O: 10%, Ar: 69.8%. (b) Gas composition: CH4: 0.2%, O2: 5%, NO: 0.15%, H2O: 10%, Ar: 69.8%. Flow rate of the mixture: 200 ml min−1, amount of catalyst: 200 mg. Figure 9: Catalytic performance of NiCo 2 O 4 in mixture of gases of exhaust of engines of natural gas vehicles. ( a ) Gas composition, CH 4 : 0.2%, O 2 : 5%, CO 2 : 15%, H 2 O: 10%, Ar: 69.8%. ( b ) Gas composition: CH 4 : 0.2%, O 2 : 5%, NO: 0.15%, H 2 O: 10%, Ar: 69.8%. Flow rate of the mixture: 200 ml min −1 , amount of catalyst: 200 mg. Full size image Crystal structures The NiCo 2 O 4 crystal structure was built by substituting Ni with Co in Co 3 O 4 crystal structure. As shown in Fig. 10 , three different substitution models of crystals were tested in our calculations, namely substituting two Co 3+ with two Ni 3+ (type I, Fig. 10a ), substituting one Co 3+ and one Co 2+ with one Ni 3+ and one Ni 2+ , respectively (type II, Fig. 10b ), and two Co 2+ with two Ni 2+ (type III, Fig. 10c ). The type I crystal structure was found to be the most stable in our calculations, while the type II was slightly less stable by 0.01 eV per unit cell higher in energy. The type III was most unfavourable thermodynamically, 0.20 eV higher per unit cell than that of type I. In the following calculations, types I and II were considered. 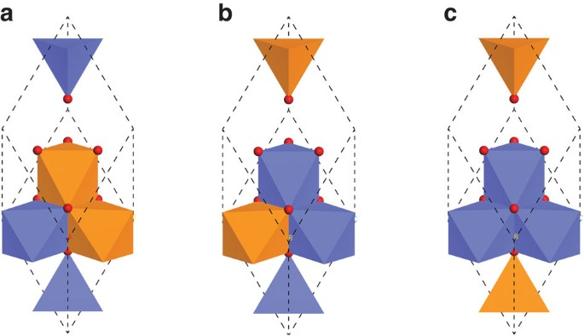Figure 10: Primitive cells of three different NiCo2O4crystals. Nickel, cobalt and oxygen are shown in orange, blue and red, respectively. (a) Two Co3+cations are substituted with two Ni3+. (b) One Co3+and one Co2+cations are substituted with one Ni3+and one Ni2+, respectively. (c) Two Co2+cations are substituted with two Ni2+. Figure 10: Primitive cells of three different NiCo 2 O 4 crystals. Nickel, cobalt and oxygen are shown in orange, blue and red, respectively. ( a ) Two Co 3+ cations are substituted with two Ni 3+ . ( b ) One Co 3+ and one Co 2+ cations are substituted with one Ni 3+ and one Ni 2+ , respectively. ( c ) Two Co 2+ cations are substituted with two Ni 2+ . Full size image Stabilities of different facets Four different surfaces namely NiCo 2 O 4 (100), NiCo 2 O 4 (110)-A, NiCo 2 O 4 (110)-B and NiCo 2 O 4 (111), were chosen for both type I and type II crystals based on the X-ray diffraction results and our previous work on Co 3 O 4 (ref. 29 ). The optimized structures were shown in Supplementary Fig. 11 and Supplementary Fig. 12 . The surface energies of all the eight surfaces were listed in Supplementary Table 1 . For both type I and type II crystals, (110)-A and (110)-B surfaces exhibit slightly higher surface energies by 0.02 or 0.03 eV than (100). (110)-A, (110)-B, and (100) of types I and II crystals with relatively low surface energies were considered in the following studies of surface reactivities. Reactivities of different facets To examine the reactivities of (110)-A, (110)-B, and (100) of type I and II crystals, the dissociations of the first C–H of CH 4 on these surfaces were investigated. Activation energies of these dissociations were listed in Supplementary Table 2 . Transition states for these dissociations were presented in Supplementary Fig. 13 and Supplementary Fig. 14 . These calculations ( Supplementary Table 2 ) suggest that the 110-B of type I crystal are the most active for CH 4 activation on Ni 3+ with lowest activation energy of only 0.52 eV which is lower than those on Ni(111) (0.88 eV) [30] , Ni(211) (0.61 eV) [30] and Pd(100) (0.79 eV) [31] . Therefore, the low barrier on 110-B of type I crystal is responsible for the high reactivity of NiCo 2 O 4 catalyst. Active sites for dissociation of the first C–H of CH 4 To assign the sites for dissociation of CH 4 to CH 3 , the binding strengths of CH 3 on cobalt and nickel sites of NiCo 2 O 4 (110)-B surfaces of both type I and type II crystals were calculated ( Supplementary Table 3 ). The adsorption energies of CH 3 on nickel sites of (110)-B are stronger than those on cobalt sites for both types of crystals. In addition, as shown in Supplementary Table 2 the activation barrier for dissociation of CH 4 to CH 3 on Ni 3+ of the most active surface NiCo 2 O 4 (110-B) of crystal type I is much lower than Co 3+ of this surface. These DFT calculations suggest that Ni 3+ cations are the sites for activating the first C–H of CH 4 . This is consistent with experimental observation. In situ studies of Ni 0.75 Co 2.25 O 4− x and Ni 1.25 Co 1.75 O 4− x with AP-XPS were performed under the same catalytic condition as NiCo 2 O 4− x . In these parallel experiments, the atomic fraction of Ni cations to the total of Ni and Co cations on the catalyst surface during catalysis was measured. As shown in Supplementary Fig. 15 , the actual fractions of Ni cations on surfaces of Ni 0.75 Co 2.25 O 4− x , NiCo 2 O 4− x , and Ni 1.25 Co 1.75 O 4− x are 0.33, 0.51 and 0.44 at 250 °C, respectively. The conversions on Ni 0.75 Co 2.25 O 4− x , Ni 1 Co 2 O 4− x , and Ni 1.25 Co 1.75 O 4− x at 275 °C are 10%, 27% and 17% ( Supplementary Figure 16 ), respectively. The correlation between atomic fractions of Ni cations in Supplementary Fig. 15 and the catalytic conversion presented in Supplementary Fig. 16 shows that a higher atomic fraction of Ni cations on surface of a Ni x Co 3− x O 4 catalyst offers higher conversion of CH 4 . It further suggests that Ni cations instead of Co cations are active sites for activating C–H of CH 4 . Mechanism of complete oxidation of CH 4 on NiCo 2 O 4 To fully understand the mechanism of CH 4 complete oxidation on NiCo 2 O 4 , a systematic investigation of potential reaction pathways was carried out on the most active surface, (110-B) of type I crystal of NiCo 2 O 4 . After the dissociation of CH 4 to CH 3 , there are two different possibilities for the next elementary steps: a further dissociation of CH 3 into CH 2 (called dehydrogenation in Supplementary Fig. 17 ) or a coupling of carbon atom of CH 3 with oxygen atom of surface lattice (called oxidation in Supplementary Fig. 17 ). In order to determine which step is more favourable, we calculated the activation energies and enthalpy change for the two potential steps. The calculated energy profiles and the corresponding geometries were shown in Supplementary Fig. 17 . Upon the first C–H dissociation, CH 3 species is oxidized into CH 3 O binding to a Ni cation. The thermodynamically and kinetically favourable oxidation step forms an intermediate, CH 3 O. This is different from the continuous dehydrogenation of CH 3 on Pd surface [14] . This preference of oxidation to CH 3 O instead of further dehydrogenation to CH 2 or CH species could be understood as follows: the low coordinated species, such as CH 2 or CH, need more than one binding sites to stabilize them; however the singly dispersed nickel cations on surface lattice of Co 3 O 4 are not an adsorption site consisting of continuously packed Ni atoms for CH 2 or CH. Therefore, a further dehydrogenation of CH 3 to CH 2 to CH is a high endothermic step on NiCo 2 O 4 compared with the pathway of oxidation. Supplementary Figure 18 presents the two potential reaction pathways A and B after the formation of CH 3 O species. DFT calculations show that pathway B is the preferred one. The following section will describe this preferred pathway. On the basis of the experimental results and previous calculations [29] , [32] , CHO species plays very important roles in the oxidation of methane on many different catalyst surfaces; thus CH 3 O could dehydrogenate to CH 2 O and then CHO with a following oxidation to form product molecules. For dehydrogenation of CH 3 O to CHO, there are two different dehydrogenation pathways schematically shown in Supplementary Fig. 18 : (i) the dehydrogenation of CH 3 O by the OH species of nickel site (pathway A shown in red in Supplementary Fig. 18 ); (ii) the dehydrogenation by the O species of nearby cobalt site (pathway B shown in black in Supplementary Fig. 18 ). On the basis of the energy profiles of the two pathways in Supplementary Fig. 19a , pathway B is more favourable than pathway A, which suggests that the dehydrogenation of CH 3 O by oxygen atoms (not shown) bonded to nearby cobalt site (pathway B) is preferred over a dehydrogenation of CH 3 O by OH species bonded to nickel site ( Supplementary Fig. 18 ) in the overall reaction (pathway A). Transformation of intermediate CHO to product molecules As mentioned above, the transformation of intermediate CHO to product molecules could go through a sub-pathway of OCHO dehydrogenation (marked with purple in the right panel of Supplementary Fig. 18 ) other than the sub-pathway of CO oxidation (marked with black in the right panel of Supplementary Fig. 18 ). Supplementary Figure 21a shows the two sub-pathways considered in our DFT calculations. Our DFT calculations revealed that each sub-pathway includes two steps with two transition states and one intermediate. OCHO is the intermediate of the sub-pathway of OCHO dehydrogenation ( Supplementary Fig. 21 ). In the sub-pathway of OCHO dehydrogenation (red in Supplementary Fig. 21a,b ), the CHO couples with oxygen atom and thus forms an intermediate OCHO (the first step in transforming CHO to product molecules); then the intermediate OCHO is dehydrogenated to CO 2 (the second step); it is quite different from the sub-pathway of CO oxidation (black line in Supplementary Fig. 21a,b ). We calculated the sub-pathway of OCHO dehydrogenation for transforming CHO to product molecules. The calculated energy profiles of the two sub-pathways were presented in Supplementary Fig. 21b . The geometries of transition states and intermediates of the sub-pathways of OCHO dehydrogenation and CO oxidation were presented in Supplementary Fig. 21c and Supplementary Fig. 21d , respectively. From the calculated energy profiles presented in Supplementary Fig. 21b , several interesting features were found. The barrier of the first transition state in the sub-pathway of OHCO dehydrogenation (red line in Supplementary Fig. 21b ) is lower than that of the first barrier in the sub-pathway of CO oxidation (black line in Supplementary Fig. 21b ); in addition, the OCHO intermediate in the sub-pathway of OCHO dehydrogenation is more thermodynamically stable than the intermediate of the sub-pathway of CO oxidation by 0.63 eV. Thus, the formation of OCHO intermediate is thermodynamically and kinetically favourable. However, the barrier for transforming OCHO intermediate to CO 2 is higher than the second barrier of the sub-pathway of CO oxidation ( Supplementary Fig. 21b ). Therefore, the formed OCHO intermediate could be experimentally observed at a relatively low temperature. In fact, our in situ studies of the catalyst surface in the mixture of CH 4 and O 2 with AP-XPS did identify the intermediate OCHO at a temperature lower than 200 °C; the C 1 s photoemission feature of this intermediate is at 288.3 eV which is consistent with the OCHO species reported in literature [25] . In addition, the observed vibration signatures of this intermediate at 1,280, 1,430, and 1,561 cm −1 in situ infrared studies ( Fig. 6 ) at 160 °C are consistent with the OCHO species formed in water–gas shift. [25] In the sub-pathway of OCHO dehydrogenation, the second step (from OCHO intermediate to product molecules shown in red line in Supplementary Fig. 21b ) is highly exothermic with a free energy change of −3.50 eV. Therefore, at high temperature the OCHO intermediate can readily overcome the barrier and transform to product molecule CO 2 , driven by the thermodynamics factor although the barrier of the second transition state is relatively high compared with the second one in the sub-pathway of CO oxidation. In fact, the evolution of C 1 s photoemission feature at 288.3 eV during catalysis from low temperature to high temperature shows that this intermediate OCHO disappears at about 200 °C along the increase of catalysis temperature ( Fig. 4d ). In situ studies using ambient pressure photoelectron spectroscopy, vibrational spectroscopy, and isotope-labelled experiments show that (1) molecular O 2 dissociates on surface oxygen vacancies; (2) the dissociated oxygen atoms fill in oxygen vacancies and couple with hydrogen atoms dissociated from intermediate to from OH and then H 2 O molecules; (3) CH 4 dissociates on Ni cations to form CH 3 with a following oxidation to CH 3 O; (4) intermediate CHO is formed through dehydrogenation of CH 3 O with oxygen species of nearby cobalt site; (5) CHO is transformed to CO 2 and H 2 O through two sub-pathways termed OCHO dehydrogenation and CO oxidation. Due to high activity and low cost of NiCo 2 O 4 catalyst in completely oxidizing CH 4 to CO 2 and H 2 O at a relatively low temperature, NiCo 2 O 4 is a very promising catalyst for removing CH 4 of gas exhaust of natural gas engine through a complete oxidation. The mechanisms of methane oxidation on NiCo 2 O 4 (100)-B are different from those on metal surfaces [14] , [30] , [32] . For instance, CH 4 on metal surfaces sequentially and continuously dehydrogenates to CH species and then is oxidized to an intermediate CHO, while our studies suggest that after dissociation of first C–H in methane, the CH 3 species will couple with oxygen atom of the lattice oxygen, forming CH 3 O species. The lack of direct dehydrogenation of CH 3 to CH 2 and then to CH on NiCo 2 O 4 likely results from the low binding energy of CH 2 or CH species on isolated Ni cations anchored on surface lattice of Co 3 O 4 . In other words, the separated Ni cation sites could not stabilize the low coordinate species such as CH 2 and CH. In these calculated pathways on the NiCo 2 O 4 (100)-B, the surface lattice oxygen atom in the nearby cobalt sites was found to be very important in the dehydrogenation of CH 3 O. Computational studies suggest that the pathways from transferring CHO to CO 2 are different from that on metal surface [14] , [33] , [34] . Sub-pathway of CO oxidation and sub-pathway of OCHO dehydrogenation were both proposed for the transformation of CHO intermediate to CO 2 . CO oxidation sub-pathway was found more kinetically favourable in the second elemental step ( Supplementary Fig. 21b ). Furthermore, the OCHO intermediate (red in Supplementary Fig. 21 ) was found to be stable at low temperature due to the high activation barrier (1.64 eV) for transforming the intermediate OCHO to product molecules. However, this intermediate (OCHO) is unstable at high temperature due to the exothermic nature of the transformation from OCHO intermediate to CO 2 ( Supplementary Fig. 21b ). Compared to the intermediate of the sub-pathway of CO oxidation, the higher thermodynamic stability of OCHO intermediate of the sub-pathway of OCHO dehydrogenation and its kinetically unfavourable transformation to CO 2 make it observable at a relatively low temperature. Synthesis NiCo 2 O 4 , Ni 1.25 Co 1.75 O 4 and Ni 0.75 Co 2.25 O 4 nanoparticles were all synthesized through a co-deposition precipitation and a following thermal decomposition. The chemicals Co(NO 3 ) 2 ·6H 2 O (≥98%), Ni(NO 3 ) 2 ·6H 2 O (≥97%), and KOH (≥85%) were purchased from Sigma-Aldrich and were used as received. 0.01 mol Ni(NO 3 ) 2 ·6H 2 O, and 0.02 mol Co(NO 3 ) 2 ·6H 2 O were physically mixed and completely dissolved in 50 ml deionized water. Then 150 ml KOH (1 M) was added under the bubbling of N 2 and with continuously stirring. During this process the temperature was kept at room temperature. A blue colloidal solution was obtained after the introduction of KOH. A dark blue precipitate was collected on centrifuging the prepared solution. Then, the dark blue precipitate was first washed with hot deionized water (60 °C) for several times with a following drying at 130 °C for 24 h. The obtained black solid was grounded to powder and was further calcined at 350 °C in air for 24 h, forming the as-synthesized catalyst NiCo 2 O 4 . To synthesize Ni 0.75 Co 2.25 O 4 and Ni 1.25 Co 1.75 O 4 , the method is almost the same as the one for the synthesis of NiCo 2 O 4. For synthesis of Ni 1.25 Co 1.75 O 4 , 0.0125, mol Ni(NO 3 ) 2 ·6H 2 O, and 0.0175, mol Co(NO 3 ) 2 ·6H 2 O were used. 0.0075, mol Ni(NO 3 ) 2 ·6H 2 O and 0.0225, mol Co(NO 3 ) 2 ·6H 2 O were used for the synthesis of Ni 0.75 Co 2.25 O 4 . Structural characterization Powder X-ray diffraction patterns of NiCo 2 O 4 , Ni 1.25 Co 1.75 O 4 , and Ni 0.75 Co 2.25 O 4 nanocatalysts were collected on a Bruker D8 advance XRD using nickel-filtered Cu Kα radiation ( λ =1.54056 Å). The measurements were operated at 40 kV and 40 mA in a continuous mode with the scanning rate of 4.2° min −1 in the 2 θ range from 10° to 80°. The size, shape and lattice fringe of catalysts were identified by high-resolution transmission electron microscope (FEI, Titan 80−300) operated at an accelerating voltage of 200 kV or lower. Image analysis was performed with Digital Micrograph (Gatan) software. The catalyst samples for TEM characterization were prepared by dropping their colloidal solutions onto copper grids supported on carbon films. In situ studies of catalysts under reaction conditions and during catalysis The in situ characterizations of surface chemistry of NiCo 2 O 4 , Ni 0.75 Co 2.25 O 4 , and Ni 1.25 Co 1.75 O 4 nanocatalysts during catalysis were performed on the in-house AP-XPS system. Monochromated Al Kα line was used as X-ray source. Unlike traditional UHV studies, in AP-XPS studies reactant gases are introduced to continuously flow through the catalyst at a desired temperature in the reaction cell while data acquisition is going on. Thus, the in situ study is defined to be a study in which the measurement of catalyst surface or adsorbate is being performed, while a catalyst is buried in gas reactant (s). The in situ characterization of AP-XPS [22] , [35] , [36] could be different from the in situ studies defined in other places since sometimes in situ study is defined as a characterization of a sample without changing location/position after a sample preparation or vapour deposition. The reaction cell was incorporated into the UHV chamber of AP-XPS system. Gas flows through the cell and exits through the exit port and an aperture that interfaces the gaseous environment in the reaction cell and vacuum environment of the prelens. Flow rate in the reaction cell was measured through a mass flow metre installed before the entrance of the reaction cell. In this study, the typical flow rate of pure gas is in the range of 3–5 ml min −1 . As the gas source used in AP-XPS studies is pure gas, 3–5 ml min −1 equals to 60–100 ml min −1 of 5% reactant gas used in catalytic measurements in a fixed-bed flow reactor. The total pressure of the mixture gas at the entrance is measured with a capacitance gauge, while the pressure at the exit is measured with another capacitance gauge. An average of the pressures at entrance and exit is defined to be the pressure above the catalyst in the reaction cell. An external heating source in the UHV environment heats the catalyst in the environment of reactant gases in the reaction cell. More detailed description of the in-house AP-XPS system can be found in our previous publications [20] . To avoid surface charging, we use Au, Ag, or HOPG to load catalysts for AP-XPS studies and control the thickness of catalyst layer on a surface [19] , [37] , [38] . In this work, we use Au foil as the substrate to physically load a thin layer of nanocatalysts. The Au foil is deliberately roughened using a SiC knife to increase the adhesion for loading. The apparent binding energies of Au 4f, Ni 2 p , Co 2 p , and O 1 s of sample prepared on the Au substrate are very close to their real values, suggesting there is no identifiable surface charging. All XPS spectra are calibrated to their corresponding Au 4f 7/2 binding energy which is at 84.0 eV. Analyses of XPS peaks are performed with Casa XPS program. In situ infrared studies are performed in a reaction cell filled with 1 bar reactant gas at Oak Ridge National Lab. This reaction cell can be heated up to high temperatures. The same catalytic condition as measurements of catalytic performances was used in the infrared studies. On-line observation of products at different temperatures Our in-house AP-XPS system also allows us to monitor the change of the gas composition during catalysis with a quadrupole mass spectrometer. Three differential pumping stages were installed between the reaction cell and the energy analyser. The aperture mounted on the reaction cell separates the high-pressure environment of the reaction cell from the vacuum of the first differential pumping stage (prelens), and also allows for leaking gases on the reaction cell into the differential pumping stages. The analyses of gas composition at different temperatures during catalysis were done by a quadrupole mass spectrometer, which is mounted at the second differential pumping stage of the AP-XPS system. To exclude the possibility that gas expansion at a high temperature or fast diffusion of molecules from reaction cell of AP-XPS to UHV chamber of mass spectrometer results in an increase of partial pressure of product molecules, Ar gas was introduced as a reference gas (background) to the reaction cell. No change in the partial pressure of Ar along with the increase of temperature of catalysts shows that the increase of partial pressure of CO 2 and H 2 O is not due to thermal expansion of gas at a relatively high temperature. Such an on-line analysis of gas composition (reactants and products) in the reaction cell of AP-XPS allows for building a simultaneous correlation between the products and real-time surface chemistry of catalysts at different catalysis temperatures. The on-line mass spectroscopy experiments allow for tracking evolution of different products at different temperatures formed through isotope-labeled catalysts or through using isotope-labelled reactant during data acquisition of in-situ AP-XPS studies. Measurements of catalytic performance The catalytic performance was measured in a fixed-bed tubular quartz micro flow reactor (inner diameter=6 mm, length=300 mm), at atmospheric pressure. The catalyst (25–500 mg) was sieved (40–60 mesh) and loaded into the reactor between two layers of quartz sands, packed in between two quartz wool plugs. The catalyst was heated in a furnace equipped with a proportional-integral-derivative temperature controller. The temperature of the catalyst was measured with a K-type thermocouple inserted into the reactor and touching the catalyst bed. The reactant gas composition was controlled by varying the flow rates of CH 4 mixture (10% CH 4 balanced in Ar) and O 2 (pure O 2 ). The flow rate of CH 4 mixture (10% balanced in Ar) and O 2 (pure) was precisely controlled through their own mass flow metres (Dakota Instruments, Inc.). When vary the flow rate of CH 4 mixture and O 2 , the ratio of pure CH 4 to pure O 2 was always keeping at 1:5. The typical flow rate of CH 4 mixture (10% balanced in Ar) is 100 ml min −1 , while the flow rate of O 2 (pure) is 50 ml min −1 . The reliability of the fix-bed reactor was checked through a blank experiment with the same experimental parameters including reactant gases, flow rate and reaction temperature. In the blank experiment, only silica supporting material was loaded in the reactor. No appreciable conversion of CH 4 was found in the blank experiment in the temperature range of 25–800 °C. The effluent gas was connected to a gas chromatograph equipped with a HayeSep D (6′ × 1/8″) packed column, a molecular sieve 13 × (6′ × 1/8″) packed column, and a thermal conductivity detector (TCD) for analysis of both reactants and products. The CH 4 conversion X% was defined as: . Herein, and are the amounts of pure CH 4 at the inlet and outlet of the reactor, respectively. In the CH 4 combustion reaction, and can be directly represented by the peak area of CH 4 in gas chromatograph before reaction and after reaction, respectively. Computational studies In this work all the DFT calculations were carried out with a periodic slab model using the Vienna ab initio simulation program [33] , [39] , [40] , [41] . The generalized gradient approximation was used with the Perdew-Burke-Ernzerhof [42] exchange-correlation functional. Due to the strong correlation effect among the partially filled Co 3 d states, we used the Hubbard parameter, U, for the Co 3 d electrons to take the on-site Coulomb interaction into account, which is the well-known DFT+U method [34] . According to previous work [29] , [43] , the value of U-J of 2 eV was applied. The projector-augmented wave method [44] , [45] was utilized to describe the electron-ion interactions, and the cut-off energy for the plane-wave basis set was 400 eV. Brillouin zone integration was accomplished using a 2 × 2 × 1 Monkhorst-Pack k-point mesh. All the adsorption geometries were optimized using a force-based conjugate gradient algorithm, while transition states were located with a constrained minimization technique [46] , [47] , [48] . How to cite this article : Tao, F. et al . Understanding complete oxidation of methane on spinel oxides at a molecular level. Nat. Commun. 6:7798 doi: 10.1038/ncomms8798 (2015).